Solar spectral conversion for improving the photosynthetic activity in algae reactors Sustainable biomass production is expected to be one of the major supporting pillars for future energy supply, as well as for renewable material provision. Algal beds represent an exciting resource for biomass/biofuel, fine chemicals and CO 2 storage. Similar to other solar energy harvesting techniques, the efficiency of algal photosynthesis depends on the spectral overlap between solar irradiation and chloroplast absorption. Here we demonstrate that spectral conversion can be employed to significantly improve biomass growth and oxygen production rate in closed-cycle algae reactors. For this purpose, we adapt a photoluminescent phosphor of the type Ca 0.59 Sr 0.40 Eu 0.01 S, which enables efficient conversion of the green part of the incoming spectrum into red light to better match the Q y peak of chlorophyll b . Integration of a Ca 0.59 Sr 0.40 Eu 0.01 S backlight converter into a flat panel algae reactor filled with Haematococcus pluvialis as a model species results in significantly increased photosynthetic activity and algae reproduction rate. Solar spectral conversion has been considered as a way to improve the efficiency of solar energy conversion processes since the early 1970s (ref. 1 ). It typically relies on a luminescence process where parts of the solar spectrum are converted to lower (downconversion, DC) [2] or higher (upconversion, UC) [3] photon energy. A net increase in conversion gain may then result from either an extension of the spectral response of the system (achievable by UC and DC) or from splitting high-energy photons into multiple photons of lower energy as long as the band-gap of the system can still be overcome (DC) [4] , [5] , [6] , [7] . UC and DC have been explored primarily for photovoltaic energy conversion where, ideally, the spectrum of incoming photons is matched to the band-gap of the employed semiconductor material. However, for various reasons (related to, for example, internal and external quantum efficiency, cost and complexity of the required module), neither DC nor UC have been technologically exploited so far. In fact, in view of additional competition from multi-junction and other improved harvesting techniques, real-world applications of DC and UC remain questionable. On the other hand, the spectral conversion of sunlight remains an intriguing tool for improving the efficiency of solar energy harvesting, when harvesting is thought beyond photovoltaic conversion. As an example, photochemical processes may be considered where the spectral response is limited to certain, comparably narrow spectral windows of the incoming light. The rate of such a reaction is proportional to the number of incident photons within the response window multiplied by the activation probability of the reaction at the respective photon energy. If the photon flux at the right photon energy is increased (and no saturation or bleaching occur), the reaction rate increases simultaneously. In principle, this can be achieved by DC and by UC in environments with low or intermediate solar irradiation intensity, to homogenize the diurnal and seasonal variation in light supply and to adjust the spectral conditions inside a flow-through reactor to a specific algae species of stage of motility. Algal beds represent one of earth’s most productive sources of biomass [8] . The high reproduction rate and large surface area make the numerous types of algae species important resources for CO 2 storage and biofuel production [9] , [10] . For example, certain algae are supposed to enable higher rates of lipid production as compared with conventional agricultural stock [11] . CO 2 -to-biomass/biofuel conversion, synthesis of fine chemicals, animal and human food fabrication, algae for cosmetics and photosynthetic gas supply are presently exploited in various stages of research and development [12] , [13] . Reactor designs reach from open ponds to km-long glass or plastic tubings to flat panels and are given significant attention [14] . As reactor designs become more efficient and applications more delicate, also light management within the reactor and at its surface becomes increasingly important [15] . When employing a luminescent spectral converter, two general designs may be considered: a frontlight converter where the incoming light is partially absorbed and converted as desired, and a backlight converter where the incoming light first passes the reactor and only the unabsorbed light participates in the conversion process before it is reflected back into the reactor containment. Both approaches have advantages and disadvantages: While apparently simple in design, the frontlight converter requires delicate management of incoming as well as secondary photons, which must not be scattered back to the atmosphere. Photons from the frontlight converter have no preferential emission direction, and thus a large fraction of photons does not enter the reaction, that is, is lost for the bio-reaction. In addition, the converter must be highly transparent for photons that are not to be converted. Both problems may be overcome in the alternative backlight converter design. The major prerequisite for a converter in backlight design is that the reactor is sufficiently transparent in the spectral range, which is to be converted to allow for enough photons to hit the converter. This sets a trade-off between maximum algae concentration, reactor thickness and converter efficiency. While this issue of scattering, reflection and residual absorption in the spectral regime of the converter can be solved by using an appropriate reactor geometry, there is no straightforward solution available today for the problem of Lambertian emission in the frontlight converter design. Here, we consider spectral conversion for improving the photosynthetic activity within an algae reactor and demonstrate that algae growth as well as oxygen production can be increased significantly by using a luminescent backlight converter, enhancing the amount of red light in the reactor. Photoluminescent converter material A schematic of the employed backlight converter design is shown in Fig. 1 . As a base phosphor material for light conversion, we have chosen strontium sulphide doped with divalent europium (SrS:Eu 2+ ), a material class commonly used in display and lighting applications [16] , [17] , [18] , [19] . Luminescence from Eu 2+ -doped materials typically occurs in a relatively broad band, which ranges from green-blue to yellow-orange, but typically does not extend far into the red. On the other hand, conversion of green light to red would be highly desirable [20] , [21] to further activate green algal chloroplasts in environments with intermediate or low solar irradiation intensity, alternatively or additively to biotechnological or biomolecular approaches [22] . For this purpose, the emission spectrum of Eu 2+ has to be pushed rather far into the red while simultaneously ensuring efficient excitation in the green. 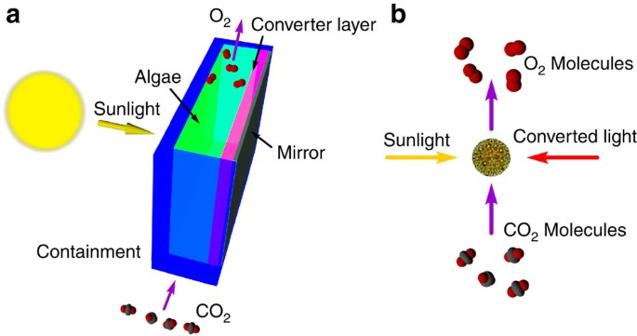Figure 1: A flat panel algae reactor combined with a solar spectral converter in backlight geometry. (a) Incoming sunlight first passes the reactor containingH. pluvialiswhere it is partially absorbed. The backside of the reactor is coated with a layer of the red-emitting phosphor Ca0.59Sr0.40Eu0.01S. The solar harvesting efficiency ofH. pluvialis—expressed as the CO2-to-biomass conversion and oxygen production rate—is improved by increasing the photon flux in the active spectral band of the algae’s chloroplasts (b). Figure 1: A flat panel algae reactor combined with a solar spectral converter in backlight geometry. ( a ) Incoming sunlight first passes the reactor containing H. pluvialis where it is partially absorbed. The backside of the reactor is coated with a layer of the red-emitting phosphor Ca 0.59 Sr 0.40 Eu 0.01 S. The solar harvesting efficiency of H. pluvialis —expressed as the CO 2 -to-biomass conversion and oxygen production rate—is improved by increasing the photon flux in the active spectral band of the algae’s chloroplasts ( b ). Full size image The photoemission spectrum of Eu 2+ arises from the d-f transition of 4f 6 5d 1 (T 2g ) to 4f 7 ( 8 S 7/2 ), where the active electronic level is not shielded against the surrounding ligands [23] . The position and width of the emission band are thus strongly dependent on the lattice the Eu 2+ -dopant is incorporated into: [24] by increasing the ligand field strength, the degree of splitting of the 4f 6 5d 1 level into the terms T 2g and E g is increased ( Fig. 2a ). This leads to a lowering of the gap between 4f 6 5d 1 ( T 2g ) and 4f 7 ( 8 S 7/2 ) and, hence, a red-shift of the photoemission band. In the present case, this increase in field strength was achieved by partially substituting Sr 2+ with Ca 2+ ions. SrS has a rock-salt structure with space group 225 (Fm m) in which Sr 2+ ions are sixfold coordinated by S 2− anions ( Fig. 2b ). It can form solid solutions with various alkaline earth, transition metal and rare earth ions at relatively high solubility [25] , [26] , [27] , [28] , [29] . Specifically, Ca 2+25 as well as Eu 2+ (ref. 30 ) can occupy Sr 2+ sites. The crystal radii of the three species (sixfold coordination) are 114, 131 and 132 pm, respectively. [31] While VI Sr 2+ and VI Eu 2+ have very similar size, VI Ca 2+ is notably smaller. It, therefore, exerts a higher field strength on its surroundings. The corresponding lattice contraction is readily visible in the X-ray diffraction patterns, Fig. 2c , where with increasing Ca 2+ -content, the diffraction peaks shift towards larger angles. From the X-ray diffraction-data, the lattice constant a was derived ( a =5.94 nm for Sr 0.75 Ca 0.25 S, a =5.87 nm for Sr 0.50 Ca 0.50 S, a =5.80 nm for Sr 0.40 Ca 0.59 Eu 0.01 S). For comparison, lattice constants of 6.02 and 5.70 nm, respectively, have been reported for single crystalline SrS and CaS (ref. 30 ). 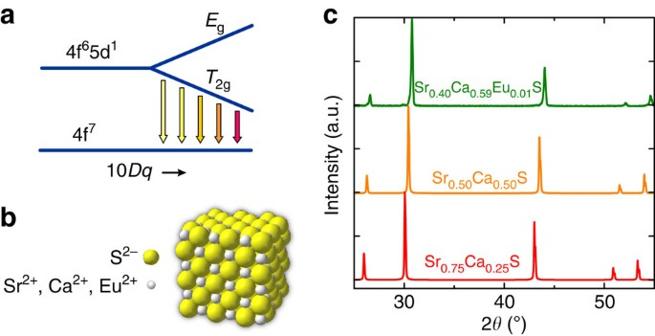Figure 2: Splitting of the 4f65d1electronic level and crystal structure in Sr1-(x+y)CaxEuyS. Electronic splitting occurs as a result of increasing crystal field strength 10Dq(a). The normalized X-ray diffraction patterns of the rock-salt structure of Sr1-(x+y)CaxEuyS (b) are shown inc. The values ofxandyare indicated in the labels. A shift of the diffraction peaks to larger angles indicates lattice contraction. a.u., arbitrary unit. Figure 2: Splitting of the 4f 6 5d 1 electronic level and crystal structure in Sr 1-( x+y ) Ca x Eu y S. Electronic splitting occurs as a result of increasing crystal field strength 10 Dq ( a ). The normalized X-ray diffraction patterns of the rock-salt structure of Sr 1-( x+y ) Ca x Eu y S ( b ) are shown in c . The values of x and y are indicated in the labels. A shift of the diffraction peaks to larger angles indicates lattice contraction. a.u., arbitrary unit. 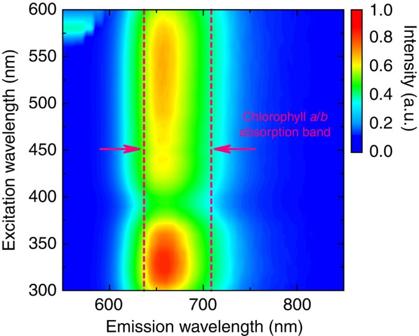Figure 3: Excitation and emission map for photoluminescence from Sr0.40Ca0.59Eu0.01S. The dashed lines are guides for the eye which indicate the position of maximal optical absorption of the considered chlorophyll species. a.u., arbitrary unit. Full size image Figure 3 depicts the excitation-emission pattern for an as-made phosphor with the optimized composition Sr 0.40 Ca 0.59 Eu 0.01 S. It consists of two broad excitation bands, which are located at ~300–380 nm and~400–590 nm, and a single emission band at ~600–750 nm. The peak of the emission band is found at 655 nm. It is practically independent on excitation wavelength. In the pure (undoped) sulphides, the ultraviolet-blue excitation band has been assigned to transitions between valence and conduction band. Although the band-gap is located at >4.3 eV (<290 nm), complex excitation schemes at energies below the band-gap have been reported for the (Ca,Sr) mixed alkaline earth sulphides [32] . On the calcium-rich side (that is, for x ~0.5...0.6), these bands have been shown to result in dominant emission at ~530 nm (ref. 32 ). The origin of the excitation bands has been related to the multiplicity of defect levels arising between valence and conduction band due to the non-statistical distribution of cations in the solid solution. Especially for the calcium-rich material and strongly dependent on synthesis procedure, this is thought to result in a relative anion deficiency [32] . In the present Eu 2+ -doped material, the gap between the two observed excitation bands is ~1.6 eV. This, on the other hand, corresponds well to the expected crystal field splitting between the 4f 6 5d 1 : T 2g and 4f 6 5d 1 : E g levels of the Eu 2+ ion ( Fig. 2 ). That is, for the single-cation sulphides SrS:Eu 2+ and CaS:Eu 2+ , splitting energies of 1.49 and 1.86 eV, respectively, have been reported [33] . While the green excitation band (400–590 nm) can readily be assigned to the 4f 7 →4f 6 5d 1 : T 2g transition of Eu 2+ , the ultraviolet-blue band can be assigned to excitation to the 4f 6 5d 1 : E g level [30] . If it is superimposed by matrix absorption as described above, due to the corresponding emission energies, energy transfer from the anion defect levels of Sr 0.40 Ca 0.59 Eu 0.01 S to 4f 6 5d 1 : T 2g in the Eu 2+ centres can be expected. Figure 3: Excitation and emission map for photoluminescence from Sr 0.40 Ca 0.59 Eu 0.01 S. The dashed lines are guides for the eye which indicate the position of maximal optical absorption of the considered chlorophyll species. a.u., arbitrary unit. Full size image Efficiency of photoconversion and reactor implementation An external quantum efficiency η EQE of (70.2±5)% was obtained for the as-prepared phosphor without further optimization or purification of raw materials ( Fig. 4 , excitation at a wavelength of 500 nm). For referencing this value, η EQE of a commercial high-performance yttrium aluminium garnet:Ce 3+ -phosphor was determined with the same experimental set-up (excitation at 450 nm, η EQE =(95.6±1)%). Photoemission from the Sr 0.40 Ca 0.59 Eu 0.01 S occurs at the CIE 1931 colour coordinates ( x ; y )=(0.69886;0.30103) (inset of Fig. 4 ), which is almost ideal red. 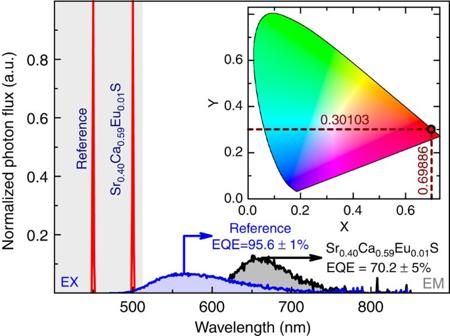Figure 4: Quantitative excitation and emission spectra for photoluminescence from Sr0.40Ca0.59Eu0.01S. The external quantum efficiency (EQE) was determined from these spectra. For comparison, the data of a reference material (commercial Ce3+-doped yttrium aluminium garnet) is included. The inset depicts the colour coordinates of the Sr0.40Ca0.59Eu0.01S photoluminescence in the CIE 1931 colour space. a.u., arbitrary unit. Figure 4: Quantitative excitation and emission spectra for photoluminescence from Sr 0.40 Ca 0.59 Eu 0.01 S. The external quantum efficiency (EQE) was determined from these spectra. For comparison, the data of a reference material (commercial Ce 3+ -doped yttrium aluminium garnet) is included. The inset depicts the colour coordinates of the Sr 0.40 Ca 0.59 Eu 0.01 S photoluminescence in the CIE 1931 colour space. a.u., arbitrary unit. Full size image The experimental implementation of the flat panel reactor design is shown in the photograph in the top part of Fig. 5 . It is further described in the Methods section. An exemplary primary solar irradiance spectrum, the resulting incoming spectrum at the backside converter after passing the reactor and the optical transmission spectrum of the reactor are shown for reference in the bottom part of Fig. 5 . In a set-up with sunlight illumination (A), the intensity spectrum of photons hitting the luminescent converter (B) is reduced because of reflection, scattering and absorption losses at the various interfaces and inside of the reactor. In particular, the optical transmission of the algae suspension (C) is largely dominated by scattering at the algae particles and chlorophyll absorption (for clarity, the absorption bands of the chloroplasts are labelled). Clearly, practically no absorption occurs in the spectral range of about 500–600 nm, and a major chlorophyll-related absorption band is found at 650–700 nm, matching-well the excitation and emission properties of the employed phosphor material. The spatial homogeneity of the phosphor layer in terms of grayscale homogeneity was ~1.4% (from 1.598.400 data points obtained at a resolution of 150 d.p.i., with an average grayscale of 170.71±2.35). 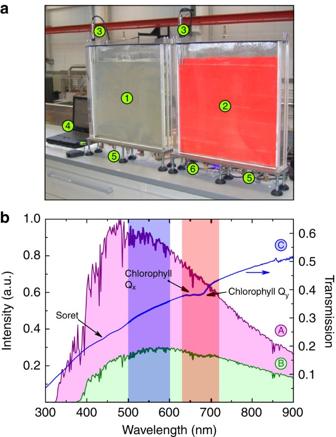Figure 5: Photograph and optical transmission data of the flat panel reactor set-up. Labels in the photograph (a) denote (1) 50 × 50 cm2reactor with backside mirror and (2) with backside converter and mirror, (3) oxygen and temperature sensors, (4) data acquisition, (5) fan pumps and (6) ultraviolet-disinfection of incoming air. Irradiance/transmittance spectra of the reactor are shown inb: (purple curve, A), as-measured solar irradiance spectrum; (green curve, B), spectrum after the light passes the reactor, but before falling onto the converter material (for 2 × 104ml−1ofH. pluvialisin active state); (C, blue curve) total transmission spectrum of the reactor before the converter material. The blue/red semitransparent vertical bars represent the absorption/emission bands of the phosphor. a.u., arbitrary unit. Figure 5: Photograph and optical transmission data of the flat panel reactor set-up. Labels in the photograph ( a ) denote (1) 50 × 50 cm 2 reactor with backside mirror and (2) with backside converter and mirror, (3) oxygen and temperature sensors, (4) data acquisition, (5) fan pumps and (6) ultraviolet-disinfection of incoming air. Irradiance/transmittance spectra of the reactor are shown in b : (purple curve, A), as-measured solar irradiance spectrum; (green curve, B), spectrum after the light passes the reactor, but before falling onto the converter material (for 2 × 10 4 ml −1 of H. pluvialis in active state); (C, blue curve) total transmission spectrum of the reactor before the converter material. The blue/red semitransparent vertical bars represent the absorption/emission bands of the phosphor. a.u., arbitrary unit. Full size image Biomass and oxygen production rate The results of algae growth and activity experiments are summarized in Figs 6 , 7 . To quantify the algae growth efficiency, we consider the total amount of biomass, expressed as the number of algae per volume. Also the oxygen production may be taken as a measure of the photosynthetic activity of H. pluvialis if it is in active state (inset in Fig. 6 ) (ref. 34 ). After an incubation time of about 4 days, significant growth activity was observed both without and in the presence of the spectral converter, that is, from about 7 × 10 4 ml −1 to a maximum of 11 × 10 4 ml −1 (without converter) and 15 × 10 4 ml −1 (with converter), respectively, after 7–8 days. This corresponds to an increase of ~36% in terms of biomass production when the converter is employed. The algae density of 11 × 10 4 ml −1 was achieved about 2 days earlier in the system, which was equipped with a backlight spectral converter. This apparent increase in efficiency is well-reproduced in the study of oxygen production rate ( Fig. 7 ). For a quantitative evaluation, we only indirectly assess the effective oxygen production rate as characteristic times after which a relative oxygen saturation of 99%, 100% and 101%, respectively, is achieved. This was done to avoid experimental misinterpretations, which might be due to oxygen loss to the air above the reactor and/or systematic variations in the flow conditions within the reactor. Data were then averaged over 12 individual cycles. When employing the spectral converter, the obtained effective saturation times were 16.6 min (for a target relative oxygen saturation of 101%), 14.3 min (100%) and 12.0 min (99%). Without converter, values of 20.2 min, 17.3 min and 14.3 min, respectively, were obtained. That is, an effective statistical increase in the oxygen production rate of ~18% was achieved. With a single exception (cycle no. 3, Fig. 7 ), an increase was observed in all experiments when employing the spectral converter. Statistical deviations between the individual cycles occur because of systematic variations of the experimental environment, especially weather conditions. 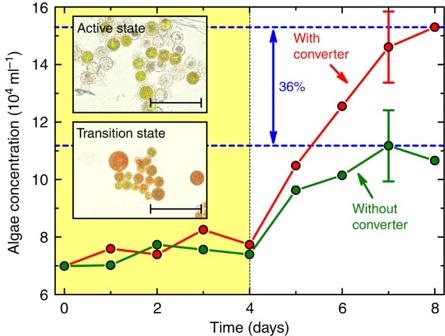Figure 6: Algae concentration as a function of time. Data represent identical reactor set-ups with (red curve) and without Sr0.40Ca0.59Eu0.01S spectral converter (green curve). The inset exemplarily shows photographs of the employed algae speciesH. pluvialisin its active and transition state. Data were obtained at room temperature in an Opticell minireactor. The yellow part of the diagram refers to the incubation time. Scale bar, 100 μm. The error bars indicate a counting error of 25,000 cells per ml. Figure 6: Algae concentration as a function of time. Data represent identical reactor set-ups with (red curve) and without Sr 0.40 Ca 0.59 Eu 0.01 S spectral converter (green curve). The inset exemplarily shows photographs of the employed algae species H. pluvialis in its active and transition state. Data were obtained at room temperature in an Opticell minireactor. The yellow part of the diagram refers to the incubation time. Scale bar, 100 μm. The error bars indicate a counting error of 25,000 cells per ml. 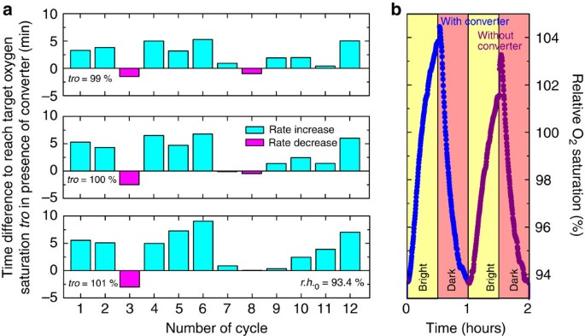Figure 7: Effect of spectral conversion on the rate of photosynthetic oxygen production. The oxygen production rate is expressed as the time after which a target relative oxygen saturationtro=99...101% is reached. Ina, the difference introwhich is obtained in the presence of a Sr0.40Ca0.59Eu0.01S spectral converter in a flat panel reactor filled withH. pluvialis(shown inFig. 5) is given. Data were obtained at room temperature for an algae concentration of ~105ml−1. Inb, the temporal change of the relative oxygen saturation is shown for an exemplary experimental cycle of 30 min bright and 30 min dark with and without converter (see text for details). Full size image Figure 7: Effect of spectral conversion on the rate of photosynthetic oxygen production. The oxygen production rate is expressed as the time after which a target relative oxygen saturation tro =99...101% is reached. In a , the difference in tro which is obtained in the presence of a Sr 0.40 Ca 0.59 Eu 0.01 S spectral converter in a flat panel reactor filled with H. pluvialis (shown in Fig. 5 ) is given. Data were obtained at room temperature for an algae concentration of ~10 5 ml −1 . In b , the temporal change of the relative oxygen saturation is shown for an exemplary experimental cycle of 30 min bright and 30 min dark with and without converter (see text for details). Full size image In conclusion, we experimentally demonstrate that green to red spectral conversion can be used to improve the energy harvesting efficiency of algal beds by >20%. Using the green algae H. pluvialis as a model system in flat panel reactors, an increase in the short-term oxygen production rate of ~18% and in the algae reproduction rate of 36% is achieved with a photoluminescent converter in backlight design under simulated solar irradiation. For this purpose, we adapted a phosphor of the type Sr 1-(x+y) Ca x Eu y S with a Sr:Ca ratio of 2:3 and an Eu 2+ doping concentration of y =0.01. This results in an optimal green to red conversion with an external quantum efficiency of >70% without further optimization. We find a splitting of about 1.55 eV between the E g and T 2g levels of Eu 2+ :4f 6 5d 1 . This leads to far red emission matching almost perfectly to the major red chloroplast absorption band of H. pluvialis . The enhancement of the number of red photons within the reactor is clearly the reason for the observed improvement in harvesting efficiency. In contrast to other schemes for improving harvesting of solar energy by spectral light conversion such as, in particular, in photovoltaic energy conversion, the present approach does not require any sophisticated technology such as transparent conductive layers, which must be compatible with the converter material. The converter material can straightforwardly be implemented into almost any reactor design. We believe that the present approach will find applications in environments with limited solar irradiance and, in particular, in closed-cycle reactors for CO 2 storage and/or synthesis of fine chemicals, where it enables improved efficiency and productivity. Phosphor synthesis and converter fabrication The Sr 0.40 Ca 0.59 Eu 0.01 S phosphor powder with a particle size range of ~1–5 μm was prepared in a solid state reaction of analytical grade CaS, SrS and Eu 2 O 3 at 1170 °C (2.5 h) in 95N 2 -5H 2 atmosphere. NH 4 Br (1.5 wt.%) and elemental sulphur (1.5 wt%) were used as flux agent and excess sulphur to account for evaporation losses, respectively. The powder morphology was analysed by scanning electron microscopy. After sedimentation in a methanol suspension and subsequent drying, the phosphor powder was mixed in a ratio of 1:2 with a commercial screen-printing lacquer (LAB-N, CoatScreen), adding 0.33 ml of dry ethanol per gram of phosphor. The phosphor-lacquer dispersion was then applied either on polyethylene-terephthalate foils or directly onto glass sheet by doctor blading, using a slit width of 200 μm and a blade speed of 10 mm per s to achieve a consolidated film thickness of (30±5) μm. The spatial homogeneity of the derived phosphor layer was evaluated via grayscale analysis of a scanned image of the layer over an area of ~20 × 30 cm. The crystal structure of the synthesized samples was analysed by powder X-ray diffractometry (X-ray diffraction, Siemens Kristalloflex D500, Bragg-Brentano, 30 kV/30 mA, Cu Kα) with a step width of 0.02° s −1 and a counting time of 10 s per step over a 2 θ range of 10–70°. Optical transmission and diffuse reflectance spectra were recorded with a dual-beam photospectrometer equipped with a 150-mm integration sphere and a PbS detector (Perkin-Elmer Lambda 950). Static photoluminescence was studied with a high-resolution spectrofluorometer (Horiba Jobin Yvon Fluorolog FL3-22) using a 450-W Xe lamp as excitation source, mechanical double monochromators in the emission and excitation channels and a red-sensitive photomultiplier tube for detection (Hamamatsu). Photoluminescence excitation spectra were corrected over the lamp intensity with a silicon photodiode and luminescence spectra were corrected by the spectral response of the detector. The external quantum efficiency η EQE of luminescence (the ratio between the numbers of emitted and absorbed photons) was obtained from three individual measurements, employing a BaSO 4 -coated integration sphere, that is, by recording the luminescence spectrum of the sample placed within the sphere, and the spectra of the sphere alone in the spectral regions of the excitation and emission of the sample. The value of η EQE was then obtained from the difference of the integrated luminescence spectra with and without sample relative to the integrated luminescence intensity, which is obtained when exciting over the complete excitation spectrum of the sphere alone. As reference, a commercial yellow phosphor, Ce 3+ -doped yttrium aluminium garnet was used. Spectral conversion and algae activity experiments As algae model, we have chosen H. pluvialis , strain no. 192.80 (provided by the Culture Collection of Algae at Goettingen University (SAG, Germany) in 2011. For the initial culture medium, we adopted the solution proposed by Fabregas [35] . In the larger flat panel reactors, algae were then suspended in natural mineral water to which 2 vol.% of a hydroponic fertilizer were added. Algae growth experiments were conducted in two types of reactors: for determining the reproduction rate in the presence and absence of the spectral converter, commercial flat minireactors with a volume of 10 ml and a lighted area of 50 cm 2 were used (OptiCell, NUNC). The reactor comprised gas-permeable membranes. Either a blank mirror or a mirror plus the converter foil were placed on the backside of the reactors ( Fig. 1 ). In order to protect the algae from eventual H 2 S evaporation from the unencapsulated phosphor layer, a thin glass sheet was placed on the backside of the reactor. Algae were counted in a Thoma chamber by extracting 300 μl of algae suspension from the reactor and adding 30 μl of ethanol to immobilize the algae. Each counting was conducted two times, and six samples were taken for each experiment. The total experimental time was chosen as a trade-off between reactor transmission and algae growth: Other than in a real-world setting where algae are constantly cycled and extracted from the reactor, our experiments represent a non-stationary state where with progressing time, the algae concentration within the reactor increases. On the one hand, this is desired to quantify the effect of the converter on the biomass production rate. On the other hand, it limits the experimental time as the optical transmission of the reactor continuously decreases and the number of photons hitting the converter is reduced, what limits the effect of the converter. This is indicated by the onset of a plateau, which can be detected in the algae concentration after about 8 days of culture. Experiments on the oxygen production rate were performed in specially constructed flat panel glass reactors with aluminium/poly-methylmethacrylate frames and silicone sealing ( Figs 1 , 5 ). Two identical reactors were used: one with a backside mirror, and one with a backside converter and mirror. The lighted area of both reactors was ~2,300 cm 2 (48 × 48 cm 2 ). The inner spacing between front and backside window was 15 mm, the total reactor volume ~3.75 l. In both series of experiments, a metal halide lamp was used as a solar simulator for constant and reproducible illumination. An infrared cutoff filter was employed to prevent heating of the reactor. Optical sensors were used to record the relative oxygen saturation and temperature in the algae suspension (Visiferm DO 120, Hamilton). pH was controlled occasionally with indicator paper. As CO 2 reservoir, ambient air was used, which was disinfected by ultraviolet-irradiation and bubbled into the reactors with a fan pump (50 l h −1 ). Measurement cycles were done at room temperature during daytime under artificial light. Each cycle comprises two alternations of 30 min of light and 30 min of dark whereby in the final minute of the dark period, converter and blank mirror were switched so that measurements with and without converter were conducted in alternations of 1 h and a total measurement cycle lasted 2 h. Here, the experimental time was chosen to ensure practically constant algae concentration. Then, the optical transmission of the reactor and the degree of converter illumination can be considered constant so that, also the effect of the converter remains constant during and between each cycle. The relative oxygen saturation through an exemplary such cycle is shown in Fig. 7b . Twelve individual such cycles were performed. The fan pump was shut-off 1 min before each light period, and restarted at the beginning of each dark period. Data were collected within 2 weeks. All experiments were done on algae in their active state (top inset in Fig. 6 ), as compared with the transition (bottom inset in Fig. 6 ) or dormant (not shown) state. How to cite this article: Wondraczek, L. et al . Solar spectral conversion for improving the photosynthetic activity in algae reactors. Nat. Commun. 4:2047 doi: 10.1038/ncomms3047 (2013).